Cryptic variation in vulva development bycis-regulatory evolution of a HAIRY-binding site Robustness to mutations is a general principle of biological systems that allows for the accumulation of cryptic variation. However, little is known about robustness and cryptic variation in core developmental pathways. Here we show through gonad-ablation screens in natural isolates of Pristionchus pacificus cryptic variation in nematode vulva development. This variation is mainly caused by cis -regulatory evolution in the conserved Notch ligand apx-1 /Delta and involves binding sites for the transcription factor HAIRY. In some isolates, including a Bolivian strain, absence of a HAIRY-binding site results in Ppa-apx-1 expression in the vulva precursor cell P6.p and causes gonad-independent vulva differentiation. In contrast, a Californian strain that gained a HAIRY-binding site lacks Ppa-apx-1 vulval expression and shows gonad-dependence of vulva development. Addition of this HAIRY-binding site to the Bolivian Ppa-apx-1 promoter eliminates expression in the vulva. Our findings indicate significant cis -regulatory evolution in a core developmental pathway leading to intraspecific cryptic variation. One of the hallmarks of the complexity of living systems is their robustness and the continued property to evolve. It has been proposed that robustness will result in cryptic variation, which provides freedom for evolutionary innovations [1] , [2] , [3] , [4] , [5] . One of the best examples for cryptic variation comes from heat-shock proteins with studies in Drosophila , Arabidopsis and yeast showing that the reduction of Hsp90 activity results in multiple morphological abnormalities [6] , [7] , [8] . Although these examples clearly indicate the buffering function of heat-shock proteins, little is known about cryptic variation in core developmental pathways and the manifestation of such variability at the micro-evolutionary level before speciation. In the nematode Pristionchus pacificus genetic studies can be coupled to natural variation [9] owing to the availability of hundreds of strains that have been recently isolated from the wild [10] , [11] . The formation of the vulva, the egg-laying structure of nematode hermaphrodites, represents an attractive system for studies on robustness and cryptic variation given the detailed knowledge and the complexity of vulval patterning mechanisms. In Caenorhabditis elegans and P. pacificus , the vulva is formed from the homologous precursor cells P(5–7).p, which are induced to have a 2°-1°-2° cell-fate pattern ( Fig. 1a ). However, vulva induction relies on different signalling input. In C. elegans EGF/RAS and LIN-12/Notch signalling act to form the robust 2°-1°-2° pattern [12] . In contrast, Wnt signalling induces vulva formation in P. pacificus [13] , [14] . Here, we show by using gonad-ablation screens in natural isolates of P. pacificus the widespread occurrence of cryptic variation in vulva development, which is to a large degree caused by cis -regulatory evolution involving a HAIRY-binding site. 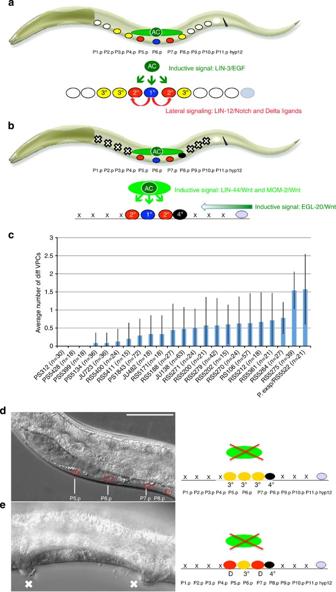Figure 1: Vulva development inC. elegansandP. pacificus. (a) Vulva formation inC. elegans. Six of 12 ventral epidermal cells generate a vulva equivalence group with P(5–7).p forming vulval tissue in wild-type animals. P6.p has the 1° fate and generates the centre of the vulva, whereas P(5,7).p have the 2° fate and form the anterior and posterior parts. The gonadal anchor cell (AC) induces vulva development by secreting the epidermal growth factor LIN-3. Cell-fate specification of P(5,7).p requires lateral LIN-12/Notch signaling from P6.p. (b) Vulva formation inP. pacificus. Seven of the 12 ventral epidermal cells die by programmed cell death (X). P(5–7).p form the vulva and have cell fates similar to those inC. elegans. However, vulva induction requires Wnt signaling and relies on redundant ligands.Ppa-EGL-20 is expressed in the posterior body region,Ppa-LIN-44 in the somatic gonad andPpa-MOM-2 in the AC, respectively. A role for lateral signaling has been deduced from cell-ablation studies, but no genetic or molecular support has been identified previously. (c) Average number of VPC differentiation after ablation of Z(1,4), the precursor cells of the somatic gonad, at the time of hatching in 22 different isolates ofP. pacificusand its sister speciesP. exspectatus.Nequals number of scored VPCs. Error bars denote s.d. (d) After Z(1,4) ablation inP. pacificusPS312/CA, VPCs do not divide and remain epidermal (yellow ovals in schematic). (e) After Z(1,4) ablation inP. pacificusRS5275/BOL, VPCs divide and form vulva-like protrusions (red ovals in schematic). Scale bar, 50 μm (ford,e). Figure 1: Vulva development in C. elegans and P. pacificus . ( a ) Vulva formation in C. elegans . Six of 12 ventral epidermal cells generate a vulva equivalence group with P(5–7).p forming vulval tissue in wild-type animals. P6.p has the 1° fate and generates the centre of the vulva, whereas P(5,7).p have the 2° fate and form the anterior and posterior parts. The gonadal anchor cell (AC) induces vulva development by secreting the epidermal growth factor LIN-3. Cell-fate specification of P(5,7).p requires lateral LIN-12/Notch signaling from P6.p. ( b ) Vulva formation in P. pacificus . Seven of the 12 ventral epidermal cells die by programmed cell death (X). P(5–7).p form the vulva and have cell fates similar to those in C. elegans . However, vulva induction requires Wnt signaling and relies on redundant ligands. Ppa -EGL-20 is expressed in the posterior body region, Ppa -LIN-44 in the somatic gonad and Ppa -MOM-2 in the AC, respectively. A role for lateral signaling has been deduced from cell-ablation studies, but no genetic or molecular support has been identified previously. ( c ) Average number of VPC differentiation after ablation of Z(1,4), the precursor cells of the somatic gonad, at the time of hatching in 22 different isolates of P. pacificus and its sister species P. exspectatus . N equals number of scored VPCs. Error bars denote s.d. ( d ) After Z(1,4) ablation in P. pacificus PS312/CA, VPCs do not divide and remain epidermal (yellow ovals in schematic). ( e ) After Z(1,4) ablation in P. pacificus RS5275/BOL, VPCs divide and form vulva-like protrusions (red ovals in schematic). Scale bar, 50 μm (for d , e ). Full size image Uncovering cryptic variation in vulva development Vulva induction in P. pacificus depends on Wnt signalling from two spatially distinct signalling centres and involves redundant mechanisms. Double and triple Wnt-pathway mutants result in a vulvaless phenotype, showing a role for the Wnt ligands Ppa-egl-20 , which is expressed in several cells in the posterior body region, and Ppa-mom-2 and Ppa-lin-44 in the gonadal anchor cell and somatic gonad, respectively ( Fig. 1b ) [13] , [14] . To search for cryptic variation in P. pacificus vulva induction we used an experimental cell-ablation approach in natural isolates of the species. Specifically, we performed a cell-ablation screen of 22 strains and looked for variation in vulva development after the ablation of Z(1,4), the precursors of the somatic gonad. Physical ablation of the gonad at hatching eliminates one of the two sources of Wnt signalling and thus, can identify cryptic variation that is normally masked by redundant signalling mechanisms. The P. pacificus PS312 strain from Pasadena (CA) served as the reference strain, as all previous cell ablation, genetic and genomic studies have been performed with this strain [13] , [14] , [15] , [16] . The other 21 strains show no heterochronies with regard to hatching and birth of the vulval precursor cells (VPCs); therefore, cell-ablation experiments were performed at the same time during development in all strains. PS312/CA and two additional strains show no VPC differentiation after ablation of Z(1,4), whereas all other 19 P. pacificus strains tested showed VPC differentiation ( Fig. 1c–e ). The average number of differentiating VPCs varies between 0 and 1.54 with the strain P. pacificus RS5275 from Bolivia (BOL) showing highest gonad-independent VPC differentiation ( Fig. 1c and Supplementary Data 1 ). Nearly, all of the differentiating VPCs adopt a 2° cell fate and form independent vulva-like protrusions with numbers varying from 0 to 3 in ablated animals ( Fig. 1e ). However, none of the ablated animals formed a functional vulva that would have been egg-laying positive. Also, none of the strains shows malformation of the vulva in un-ablated animals. Thus, massive cryptic variation after Z(1,4) ablation exists in P. pacificus , which is masked in un-ablated animals by gonadal signalling. Genetic basis of vulval variation in Pristionchus To study the molecular mechanisms associated with the observed natural variation in VPC differentiation, we selected PS312/CA and RS5275/BOL with their extreme phenotypes of VPC differentiation after Z(1,4) ablation, to perform recombinant inbred line (RIL) experiments. We identified a major quantitative trait locus (QTL) associated with the marker S595 on chromosome I with a LOD score of 7.7 and a smaller but still significant QTL on chromosome II with a LOD score of 3.3 ( Supplementary Fig. S1 ; Supplementary Data 2 ). Next, we constructed near-isogenic lines, which defined a 346-kb region with the breakpoints SI26069 and SI24420 on chromosome I ( Fig. 2a ; Supplementary Fig. S2 and Supplementary Data 2 , Supplementary Data 3 ). This region is physically associated with the QTL at S595 and contains 21 gene predictions ( Fig. 2a and Supplementary Table S1 ). Computational analysis identified the conserved developmental control gene Ppa-apx-1 /Delta as a potential candidate gene in this interval (WormBase PP08489) ( Fig. 2a ). The Delta gene family encodes for ligands of the LIN-12/Notch receptors and is conserved throughout the animal kingdom [17] . Ten genes of the Delta/Serrate/Lag-2 (DSL) family exist in C. elegans . Ppa-apx-1 is most similar to Cel-apx-1 and contains a DSL domain, four EGF (epidermal growth factor) domains, and a transmembrane domain ( Fig. 2a ). Cel-apx-1 is expressed in P6.p and was shown to mediate lateral signalling from P6.p to P(5,7).p in a redundant manner with two other Delta family members, Cel-dsl-1 and Cel-lag-2 ( [17] ). In P. pacificus , lateral signalling between VPCs is anticipated based on cell-ablation studies [16] , but no genetic evidence has been obtained from saturated mutagenesis screens. 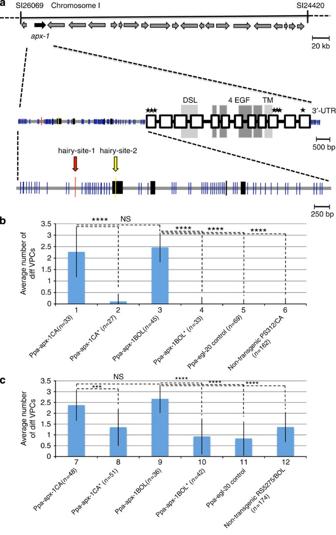Figure 2:Ppa-apx-1genome location and transgenes. (a) Row 1:Ppa-apx-1is located in a 346-kb region of chromosome I, which contains 21 gene predictions (arrows). For a full list of genes seeSupplementary Table S2. Row 2:Ppa-apx-1gene structure and comparison between PS312/CA and RS5275/BOL.Ppa-apx-1has 12 exons (rectangles) and contains a conserved Delta/Serrate/LAG-2 (DSL) domain, four epidermal growth factor (EGF) domains, and a transmembrane (TM) domain, all shown in different shading. Asterisks denote polymorphisms or indels that result in amino-acid substitutions between PS312/CA and RS5275/BOL. Row 3: A 5-kb promoter region contains multiple single-nucleotide polymorphisms and small, insertions/deletions (blue) and three larger elements with few sequence similarities (black bars). The PS312/CAPpa-apx-1promoter contains two HAIRY-binding sites, hairy-site-1 is found in PS312/CAL, RS5275/BOL, as well as other strains (red line). Hairy-site-2 is found only in PS312/CA and a few other strains (yellow line) and is located in a region without sequence similarity betweenPpa-apx-1CAandPpa-apx-1BOL. For a detailed description of RILs and NILs, seeSupplementary Data 2andSupplementary Table S4. (b) Gonad ablation of transgenic animals and control animals in a PS312/CA background. Experimental setups are numbered 1–6. Transgenic lines carrying either aPpa-apx-1CA(1) orPpa-apx-1BOL(3) transgene both show gonad-independent vulva differentiation in >75% of the VPCs (2 out of the 3 VPCs). Control animals are either non-transgenic sisters (*) that have lost the transgenic array of both constructs (2,4),Ppa-egl-20::RFP transgenic animals (5), or PS312/CA wild-type animals (6). All controls show <5% gonad-independent differentiation. (c) Gonad ablation of transgenic animals in the RS5275/BOL background. Experimental setups are numbered 7–12. Transgenic lines carrying either aPpa-apx-1CA(7) orPpa-apx-1BOL(9) transgene both show gonad-independent vulva differentiation in more than two out of the three VPCs on average. Control animals show gonad-independent differentiation in 30–60% of the VPCs according to the RS5275/BOL genetic background. Controls include non-transgenic sisters (*) that have lost the transgenic array of both constructs (8,10),Ppa-egl-20::RFP transgenic animals (11), or RS5275/BOL wild-type animals (12). Error bars denote standard deviation. ***P<0.001, ****P<0.0001 (two samplet-test). A detailed description of constructs and ablation results is provided asSupplementary Tables S2 and S3. Figure 2: Ppa-apx-1 genome location and transgenes. ( a ) Row 1: Ppa-apx-1 is located in a 346-kb region of chromosome I, which contains 21 gene predictions (arrows). For a full list of genes see Supplementary Table S2 . Row 2: Ppa-apx-1 gene structure and comparison between PS312/CA and RS5275/BOL. Ppa-apx-1 has 12 exons (rectangles) and contains a conserved Delta/Serrate/LAG-2 (DSL) domain, four epidermal growth factor (EGF) domains, and a transmembrane (TM) domain, all shown in different shading. Asterisks denote polymorphisms or indels that result in amino-acid substitutions between PS312/CA and RS5275/BOL. Row 3: A 5-kb promoter region contains multiple single-nucleotide polymorphisms and small, insertions/deletions (blue) and three larger elements with few sequence similarities (black bars). The PS312/CA Ppa-apx-1 promoter contains two HAIRY-binding sites, hairy-site-1 is found in PS312/CAL, RS5275/BOL, as well as other strains (red line). Hairy-site-2 is found only in PS312/CA and a few other strains (yellow line) and is located in a region without sequence similarity between Ppa-apx-1 CA and Ppa-apx-1 BOL . For a detailed description of RILs and NILs, see Supplementary Data 2 and Supplementary Table S4 . ( b ) Gonad ablation of transgenic animals and control animals in a PS312/CA background. Experimental setups are numbered 1–6. Transgenic lines carrying either a Ppa-apx-1 CA (1) or Ppa-apx-1 BOL (3) transgene both show gonad-independent vulva differentiation in >75% of the VPCs (2 out of the 3 VPCs). Control animals are either non-transgenic sisters (*) that have lost the transgenic array of both constructs (2,4), Ppa-egl-20:: RFP transgenic animals (5), or PS312/CA wild-type animals (6). All controls show <5% gonad-independent differentiation. ( c ) Gonad ablation of transgenic animals in the RS5275/BOL background. Experimental setups are numbered 7–12. Transgenic lines carrying either a Ppa-apx-1 CA (7) or Ppa-apx-1 BOL (9) transgene both show gonad-independent vulva differentiation in more than two out of the three VPCs on average. Control animals show gonad-independent differentiation in 30–60% of the VPCs according to the RS5275/BOL genetic background. Controls include non-transgenic sisters (*) that have lost the transgenic array of both constructs (8,10), Ppa-egl-20:: RFP transgenic animals (11), or RS5275/BOL wild-type animals (12). Error bars denote standard deviation. *** P <0.001, **** P <0.0001 (two sample t -test). A detailed description of constructs and ablation results is provided as Supplementary Tables S2 and S3 . Full size image Ppa-apx-1 /Delta as major determinant for cryptic variation To test whether Ppa-apx-1 is indeed the causative gene for the major QTL we generated transgenic animals in cis- and trans- configurations. The coding region of Ppa-apx-1 in PS312/CA and RS5275/BOL contains 18 single-nucleotide polymorphisms and 7 small indels that result in a total of seven amino-acid substitutions, all of which are conservative and none of which causes a frame shift or is located in a functional domain of the protein ( Fig. 2a ). In contrast, we identified more than 50 single-nucleotide polymorphisms and 30 indels in a 5-kb promoter area of Ppa-apx-1 ( Fig. 2a ). We constructed transgenic animals in which a 12.5-kb genomic construct containing a 5-kb promoter region, the coding region, and the 3′-UTR of Ppa-apx-1 were injected into both strains. Surprisingly, transgenic lines of all four possible combinations showed a strong transgression phenotype after Z(1,4) ablation ( Fig. 2b and Supplementary Tables S2, S3 ). Specifically, more than two of the three VPCs showed vulva differentiation on average after Z(1,4) ablation in transgenic lines containing Ppa-apx-1 CA or Ppa-apx-1 BOL in the PS312/CA and the RS5275/BOL background, respectively. These results strongly suggest that Ppa-apx-1 is the gene causing the major QTL for cryptic variability in vulva formation. Furthermore, these data provide evidence that Ppa-apx-1 function is dosage-dependent because overexpression of either form of the gene in both natural backgrounds causes a VPC differentiation phenotype after gonad ablation. Also, VPC differentiation in transgenic animals is stronger than what is observed in natural isolates. Differential expression of Ppa-apx-1 in vulval cells To further investigate the function of Ppa-apx-1, we studied the expression of Ppa-apx-1 CA and Ppa-apx-1 BOL using transcriptional reporters. Ppa-apx-1 BOL is expressed in P6.p, starting early in the J3 stage and continuing until the late J4 stage in the progeny of P6.p ( Fig. 3a ). Ppa-apx-1 BOL is also specifically expressed in several ventral neurons and in an unidentified lateral neuron ( Supplementary Fig. S4 ). In contrast, there is no expression of Ppa-apx-1 CA in P6.p or any other vulval cell ( Fig. 3b ). We generated four independent lines from two distinct reporter constructs of Ppa-apx-1 CA , none of which shows expression in P6.p and ventral neurons. However, Ppa-apx-1 CA expression is present in the same lateral neuron as observed for Ppa-apx-1 BOL , suggesting that the constructs are functional ( Supplementary Fig. S4 ). Interestingly, the Ppa-apx-1 BOL construct shows RFP expression in a similar manner in the RS5275/BOL and the PS312/CA strain indicating that distinct cis -regulatory elements are responsible for the observed differences in vulval expression ( Fig. 3a ). We conclude that Ppa-apx-1 CA and Ppa-apx-1 BOL differ from each other with respect to their expression in vulva development. Two specific hypotheses follow from these results. First, expression of Ppa-apx-1 BOL suggests an instructive role in lateral signalling from P6.p to P(5,7).p, which might depend on Wnt signalling. Second, the absence of Ppa-apx-1 CA expression in P6.p might indicate that Ppa-apx-1 -based lateral signalling has either been lost or strongly reduced in the PS312/CA strain. 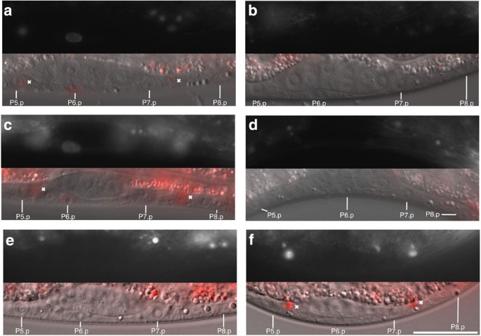Figure 3: Expression pattern analysis ofPpa-apx-1in different genetic backgrounds. (a) Early J3 stage of a RS5275/BOL animal carrying a 6-kb transcriptional reporter construct. ThePpa-apx-1BOLconstruct shows RFP expression in P6.p and in some ventral neurons surrounding P5.p and P7.p (crosses). (b) Early J3 stage of a PS312/CA animal carrying a similar transcriptional reporter construct ofPpa-apx-1CA. There is no RFP expression in P6.p and ventral neurons. (c) A PS312/CA animal carrying thePpa-apx-1BOLreporter construct shows RFP expression in P6.p and ventral neurons. (d) ThePpa-apx-1CAreporter construct shows no RFP expression in P6.p and ventral neurons in the RS5275/BOL background. (e) APpa-apx-1BOLconstruct with an inserted California hairy-site-2 does not show RFP expression in P6.p and ventral neurons. (f) APpa-apx-1CAconstruct with a deleted hairy-site-2 shows RFP expression in ventral neurons (crosses), but shows no RFP expression in P6.p. Expression patterns are based on at least five animals per age group (early/mid/lateJ2, J3 J4 and adult) and were totally consistent between animals. Pictures were taken using the same microscope settings. Reddish background is based on auto-fluorescence in the gut. Scale bar, 20 μm. Figure 3: Expression pattern analysis of Ppa-apx-1 in different genetic backgrounds. ( a ) Early J3 stage of a RS5275/BOL animal carrying a 6-kb transcriptional reporter construct. The Ppa-apx-1 BOL construct shows RFP expression in P6.p and in some ventral neurons surrounding P5.p and P7.p (crosses). ( b ) Early J3 stage of a PS312/CA animal carrying a similar transcriptional reporter construct of Ppa-apx-1 CA . There is no RFP expression in P6.p and ventral neurons. ( c ) A PS312/CA animal carrying the Ppa-apx-1 BOL reporter construct shows RFP expression in P6.p and ventral neurons. ( d ) The Ppa-apx-1 CA reporter construct shows no RFP expression in P6.p and ventral neurons in the RS5275/BOL background. ( e ) A Ppa-apx-1 BOL construct with an inserted California hairy-site-2 does not show RFP expression in P6.p and ventral neurons. ( f ) A Ppa-apx-1 CA construct with a deleted hairy-site-2 shows RFP expression in ventral neurons (crosses), but shows no RFP expression in P6.p. Expression patterns are based on at least five animals per age group (early/mid/lateJ2, J3 J4 and adult) and were totally consistent between animals. Pictures were taken using the same microscope settings. Reddish background is based on auto-fluorescence in the gut. Scale bar, 20 μm. Full size image Genetic interaction of Ppa-apx-1 and Wnt signalling To test these hypotheses, we first looked for genetic interactions between Ppa-apx-1 and Wnt signalling. We crossed the Ppa-apx-1 BOL reporter construct into the Ppa-bar-1(tu362) /β-catenin mutant, which has a strong Vulvaless phenotype, because it interferes with Wnt signalling from both the gonad and the posterior body region [13] , [14] . We found that Ppa-apx-1 BOL expression is absent from P6.p in Ppa-bar-1(tu362) /β-catenin mutants, indicating that Ppa-apx-1 BOL expression is Wnt-signalling dependent ( Fig. 4a ). Next, we analysed Ppa-apx-1 BOL expression in gonad-ablated animals and found that it is still weakly expressed in P6.p ( Supplementary Fig. S3 ). These results suggest that the ablation of the gonad eliminates a major, but not the complete Wnt signalling, input regulating Ppa-apx-1 BOL expression in P6.p. 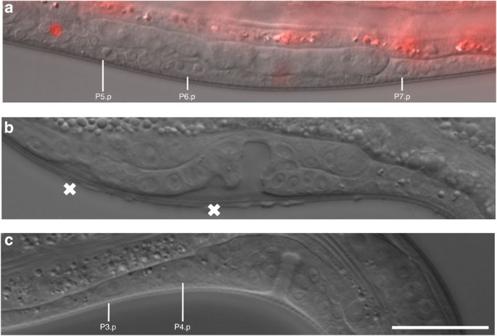Figure 4: Expression pattern analysis and overexpression ofPpa-apx-1in different mutant backgrounds. (a) Mid J4 stage of aPpa-bar-1(tu362)mutant animal carrying a 6-kb transcriptional reporter construct ofPpa-apx-1BOLshows no RFP expression in P6.p. (b) Overexpression ofPpa-apx-1BOLinPpa-hairy(sy344)mutants results in vulva differentiation of P(3,4).p (X) anterior to the normal vulva (Multivulva phenotype). (c) APpa-ced-3(tu54)mutant carrying the same transgene as in (b) does not cause differentiation of P(3,4).p. All analyses are based on at least 20 animals. Scale bar, 20 μm. Figure 4: Expression pattern analysis and overexpression of Ppa-apx-1 in different mutant backgrounds. ( a ) Mid J4 stage of a Ppa-bar-1(tu362) mutant animal carrying a 6-kb transcriptional reporter construct of Ppa-apx-1 BOL shows no RFP expression in P6.p. ( b ) Overexpression of Ppa-apx-1 BOL in Ppa-hairy(sy344) mutants results in vulva differentiation of P(3,4).p (X) anterior to the normal vulva (Multivulva phenotype). ( c ) A Ppa-ced-3(tu54) mutant carrying the same transgene as in ( b ) does not cause differentiation of P(3,4).p. All analyses are based on at least 20 animals. Scale bar, 20 μm. Full size image Binding sites for HAIRY in the Ppa-apx-1 promoter Next, we wanted to determine if differences in the cis -regulatory elements of the Ppa-apx-1 CA and Ppa-apx-1 BOL promoters are responsible for the differences in expression. Interestingly, we found that a 150-bp region in the promoter of Ppa-apx-1 CA contains a bonafide binding site for the transcription factor HAIRY, which is absent from Ppa-apx-1 BOL (hairy-site-2 in Fig. 2a ). Another HAIRY-binding site is present in both promoters (hairy-site-1 in Fig. 2a ). Thus, Ppa-apx-1 CA contains two but Ppa-apx-1 BOL contains only one HAIRY-binding site. HAIRY-related proteins are members of the basic helix-loop-helix family of transcription factors that have been shown to act as repressors in cell-fate decisions as well as effectors for Notch signalling in Drosophila and vertebrates [18] , [19] . During P. pacificus vulva development, Ppa-hairy regulates the size of the vulva equivalence group by repressing the activity of the Hox gene lin-39 ( [20] ). In Ppa-hairy mutants, the two anterior epidermal cells P(3,4).p do not undergo programmed cell death as they do in wild-type animals. Rather, they survive and remain epidermal, which makes them competent to adopt a vulval fate under certain experimental or mutant conditions [20] . Although hairy is conserved throughout the animal kingdom, C. elegans has lost the hairy gene in its recent evolutionary history [20] . Ppa-HAIRY functions as repressor for Ppa-apx-1 One potential role of Ppa -HAIRY could be the repression of Ppa-apx-1 expression in P6.p in PS312/CA. Presence of two HAIRY-binding sites in the Ppa-apx-1 CA promoter might result in the absence or strong reduction of expression in P6.p and gonad-dependence of vulva differentiation. In contrast, the absence of hairy-site-2 in Ppa-apx-1 BOL might allow Ppa-apx-1 expression in P6.p, resulting in Wnt-dependent lateral signalling and gonad-independent vulva differentiation. To test this hypothesis, we performed two types of experiments. First, we crossed the Ppa-apx-1 BOL transgene into Ppa-hairy(sy344) mutant animals. Indeed, we observed a strong Multivulva phenotype and cell lineage analysis indicated that P(3,4).p adopted a 2° cell fate ( Fig. 4b ). Although these findings are in agreement with the repression of Ppa-apx-1 expression by Ppa-hairy , they cannot directly rule out that the survival of P(3,4).p in Ppa-hairy mutants alone causes the Multivulva phenotype in Ppa-apx-1 transgenic backgrounds. Therefore, we crossed the Ppa-apx-1 BOL transgene into the Ppa-ced-3(tu54) mutant, in which P(3,4).p also survive because of a general cell-death defect [21] . In the Ppa-ced-3(tu54) background Ppa-apx-1 BOL transgenes do not cause a Multivulva phenotype ( Fig. 4c ). These results suggest that Ppa -HAIRY functions as a repressor of Ppa-apx-1 expression. Additional experiments indicate that Ppa-apx-1 expression in the Ppa-hairy(sy344) mutant background is similar to wild-type. Although Ppa-hairy mutants carrying a Ppa-apx-1 CA reporter construct do not show RFP expression in P6.p, Ppa-hairy mutants carrying a Ppa-apx-1 BOL reporter construct show a stronger RFP expression compared to wild-type animals, but not in additional vulval cells ( Supplementary Fig. S5 and Fig. 3a ). Together, these findings are consistent with the idea that Ppa-apx-1 can act over a distance. HAIRY-site-2 is necessary to prevent Ppa-apx-1 expression In a second set of experiments, we engineered modified cis -regulatory elements of Ppa-apx-1 in order to directly study the involvement of the presence or absence of the hairy-site-2 in P6.p expression of Ppa-apx-1 . Indeed, we could show that the insertion of the second HAIRY-binding site into the Ppa-apx-1 BOL promoter resulted in the absence of Ppa-apx-1 expression in P6.p ( Fig. 3e ). This result suggests that this HAIRY-binding site is necessary to prevent Ppa-apx-1 expression in P6.p. Next, we eliminated the hairy-site-2 from the Ppa-apx-1 CA reporter. Animals carrying this construct showed a gain of RFP expression in those ventral neurons that are also expressed in animals carrying the Ppa-apx-1 BOL reporter constructs ( Fig. 3f ). However, there is no RFP expression in P6.p ( Fig. 3f ), indicating that additional regulatory elements in the promoter are involved in the regulation of Ppa-apx-1 in P6.p in the Californian strain. Evolution of HAIRY-binding sites in the Ppa-apx-1 promoter The overall pattern of gonad-independent vulva differentiation in different wild isolates ( Fig. 1c ) would be consistent with the idea that the hairy-site-2 in the Ppa-apx-1 CA promoter is a recent evolutionary invention. To test this idea, we used phylogenetic footprinting based on computational analysis. We identified hairy-site-2 in RS5428 and RS5399 from La Réunion, the two strains that show no gonad-independent vulva differentiation, similar to PS312/CA ( Fig. 1c and Supplementary Table S4 ). Similarly, two more strains with <5% VPC differentiation (RS5134, RS5400) also contain hairy-site-2 in their Ppa-apx-1 promoters. This strong correlation did not hold true for strains showing an intermediate gonad-ablation phenotype arguing that additional regulatory elements are present, which have yet to be identified. Alternatively, other genes might be involved in the gonad-independent VPC differentiation as already indicated by the second QTL peak in the PS312/CA—RS5275/BOL RILs ( Supplementary Fig. S1c ). To provide further support for the hypothesis that hairy-site-2 is a recent evolutionary invention we analysed the apx-1 locus in the closely related sister species P. exspectatus as an outgroup comparison [22] . After Z(1,4) ablation, more than half of the VPCs differentiate in P. exspectatus ( Fig. 1c ). Although the apx-1 -coding region is similar between both species and hairy-site-1 is conserved, hairy-site-2 is not found in P. exspectatus ( Supplementary Table S4 ). Together, these findings are consistent with the idea that hairy-site-2 is a novel cis -regulatory element in PS312/CA representing a recent evolutionary invention. This study indicates cryptic variation in a core developmental pathway. We identified the Delta-like signalling molecule apx-1 as a major contributing locus and found changes in cis -regulatory elements resulting in cryptic variation. The Delta/Notch system represents a highly conserved signalling pathway with an enormous diversification of Delta-like ligands in C. elegans [19] . This study indicates that Ppa-apx-1 contributes to lateral signalling in vulva development, and suggests that after ablation of the gonad, Ppa-apx-1 functions in the generation of 2°-like vulva protrusions in RS5275/BOL. Based on the finding that when overexpressed as a transgene even the Ppa-apx-1 CA gene is able to induce gonad-independent vulva differentiation, we hypothesize that the levels of apx-1 required to confer gonad-independent vulva differentiation are lower than the levels required for RFP detection. This observation is similar for wild-type and Ppa-hairy mutant animals. The observed role of HAIRY as a transcriptional repressor confirms previous findings of repressor function in P. pacificus and other animals, although the HAIRY gene has been lost in C. elegans [20] . Some studies in insects revealed cis -regulatory differences between closely related species and have highlighted the importance of novel expression domains [23] , [24] , [25] . Previous work in nematodes indicated developmental differences between Pristionchus strains and species [9] and a recent study mapped natural variation in C. elegans vulva development between strains to differences in the coding region of the nath-10 gene [26] . Our study shows that significant changes in cis -regulatory elements can occur before speciation and that they can result in cryptic variation between different strains of the same biological species. This observation supports the notion that developmental mechanisms are under continuous turnover and are subject to drift. Facilitated by redundancy and developmental buffering, these types of cryptic changes can accumulate in the absence of selection and can have long-term consequences for the wiring of developmental networks. All strains used in this study were inbred for at least 10 generations and are described elsewhere [10] , [11] . Cell-ablation experiments were carried out using standard techniques [27] , by ablating the gonad 0–1 h after hatching of the larvae (20 °C). RILs were set up by crossing 3–5 males of RS5275/BOL to 1 virgin hermaphrodite of PS312/CA and heterozygous F1 animals were determined using standard mapping markers [28] ( www.pristionchus.org ). Heterozygous F1 animals were isolated and, in the F2, single animals were transferred to new plates and allowed to self-fertilize. Single-offspring larvae were randomly chosen and transferred to new plates in every generation until the F10. After 10 generation of inbreeding all RILs and NILs were expected and confirmed to be homozygous for most loci on all Chromosomes. NILs were constructed by continuously back-crossing RILs showing PS312/CA phenotype to RS5275/BOL males. RILs and NILS were phenotyped by ablation of Z(1,4). 37 evenly spaced markers were used for genotyping RILs [28] ( www.pristionchus.org ). QTL mapping of the gonad-independent VPC differentiation phenotype was carried out using the software R/qtl. Marker distances were calculated using the program R/qtl. Transgenesis experiments were performed by coinjecting a Ppa-apx-1 CA or Ppa-apx-1 BOL transgene (0.5–2 ng μl −1 ) with the marker plasmid Ppa-egl-20 /Wnt: TurboRFP (10 ng μl −1 ) and genomic carrier DNA (60 ng μl −1 ) as described previously [29] . The Ppa-apx-1 CA and Ppa-apx-1 BOL transgenes contained the entire 6 kb Ppa-apx-1- coding and non-coding region plus a 5-kb upstream and a 1.3-kb downstream region. In the expression constructs, the promoter region of Ppa-apx-1 (5 kb upstream of the start codon) was cloned into the puC19 vector containing NLS/RFP region plus rpl-23 3′-UTR. For all constructs, multiple independent lines were generated. How to cite this article: Kienle, S. & Sommer R.J. Cryptic variation in vulva development by cis -regulatory evolution of a HAIRY-binding site. Nat. Commun. 4:1714 doi: 10.1038/ncomms2711 (2013).